The transcription factor Foxc1 is necessary for Ihh–Gli2-regulated endochondral ossification Indian hedgehog (Ihh) regulates endochondral ossification in both a parathyroid hormone-related protein (PTHrP)-dependent and -independent manner by activating transcriptional mediator Gli2. However, the molecular mechanisms underlying these processes remain elusive. Here by using in vivo microarray analysis, we identify forkhead box C1 (Foxc1) as a transcriptional partner of Gli2. Foxc1 stimulates expression of Ihh target genes, including PTHrP and Col10a1, through its physical and functional interaction with Gli2. Conversely, a dominant negative Foxc1 inhibits the Ihh target gene expression. In a spontaneous loss of Foxc1 function mouse (Foxc1 ch/ch ), endochondral ossification is delayed and the expression of Ihh target genes inhibited. Moreover, the pathological Foxc1 missense mutation observed in the Axenfeld–Rieger syndrome impairs Gli2–Foxc1 association as well as Ihh function. Our findings suggest that Foxc1 is an important transcriptional partner of Ihh–Gli2 signalling during endochondral ossification, and that disruption of the Foxc1–Gli2 interaction causes skeletal abnormalities observed in the Axenfeld–Rieger syndrome. Skeletal development occurs via two independent biological processes known as intramembranous ossification and endochondral ossification [1] . During intramembranous ossification, mesenchymal stem cells differentiate into osteoblasts that produce and mineralize bone matrix without cartilage template. The clavicle and flat bones, including calvaria, mandible and maxilla, are formed by intramembranous ossification [2] , [3] . In contrast, endochondral ossification is mainly conducted by chondrocytes and involves sequential steps of chondrocyte differentiation followed by the replacement of bone [4] . During early stage chondrocyte differentiation, mesenchymal cells condense and differentiate into resting and proliferating chondrocytes that produce abundant extracellular matrix, including type-2 collagen and aggrecan [5] . In the late stage, proliferating chondrocytes become hypertrophic chondrocytes that produce type-10 collagen and matrix metalloproteinase (MMP)-13 (ref. 4 ). Finally, the hypertrophic chondrocytes undergo apoptosis, which is followed by the invasion of blood vessels and osteoblasts [6] . In humans, most long bones and some craniofacial bones, including the mandibular condyle and sphenoid bone, are formed by endochondral ossification. Thus, the impairment of endochondral ossification causes various skeletal abnormalities, including a short stature and facial dysmorphism [7] . Different cytokines, growth factors and hormones regulate endochondral ossification by activating intracellular signalling molecules and transcription factors. Bone morphogenetic protein family members control chondrocyte proliferation and matrix synthesis by activating Smads [8] , [9] ; cartilage-specific deletion of Smad1/5 in mice results in severe chondrodysplasia [10] . Indian hedgehog (Ihh), a member of the hedgehog family, plays critical roles in the endochondral ossification via its regulation of genes, such as parathyroid hormone-related protein ( PTHrP ), protein patched homologue 1 ( Ptch1 ), α1(X) collagen ( Col10a1 ) and Gli1 , by activating the transcription factor Gli2 (refs 11 , 12 , 13 , 14 ). The deletion of Ihh or Gli2 causes severe skeletal defects with reduced chondrocyte proliferation and maturation [15] , [16] , [17] . In addition, Sex-determining region Y-type high mobility group box protein 9 (Sox9) and Runt-related transcription factor 2/3 (Runx2/3), are critical transcription factors for early chondrogenesis [18] and chondrocyte hypertrophy [19] . The transcriptional machineries of individual genes assemble into transcriptional networks that orchestrate the complicated but well-organized chondrocyte differentiation steps during endochondral ossification [20] . Thus, the identification and characterization of novel transcription factors involved in these processes will contribute to a better understanding of endochondral ossification. Numerous attempts have been made to identify these and we previously identified several transcription factors using a high-throughput assay system [21] , [22] , [23] , [24] and Solexa deep-sequencing technology [25] . However, the transcriptional networks of endochondral ossification are still not fully elucidated. In this study, we established a gene-screening system to identify novel transcription factors involved in endochondral ossification using a combination of chondrocyte reporter mice and flow cytometry (fluorescence-activated cell sorting, FACS)-assisted microarray analysis. This revealed that forkhead box c1 (Foxc1) plays a critical role in endochondral ossification through its physical and functional association with Ihh–Gli2 signalling. We also established that the loss of interaction caused by a missense mutation in Foxc1 partially accounts for pathogenesis of the abnormal skeletal development observed in the Axenfeld–Rieger syndrome. Our findings provide new insights into the transcriptional network system that is critical for endochondral ossification and demonstrate a pathogenic mechanism of skeletal abnormalities in the Axenfeld–Rieger syndrome. Identification of genes selectively expressed in cartilage We first attempted to identify transcription factors that were highly expressed in developing cartilage during the embryonic stage. In particular, we aimed to isolate transcription factors relevant to the in vivo situation. We, therefore, generated transgenic mice in which the chondrocytes were fluorescently labelled with the Venus gene expression reporter driven by the Col2a1 promoter ( Col2a1 -Venus-Tg; Supplementary Fig. 1a ). Exogenous expression of Venus in cartilage tissues of Col2a1 -Venus-Tg mice was confirmed by fluorescence stereomicroscopy ( Supplementary Fig. 1b,c ). Cartilage from the limbs, rib cages and vertebrae of E13.5 Col2a1 -Venus-Tg mice was dissociated and digested into single cells using collagenase and trypsin ( Supplementary Fig. 1d ). Venus-negative and -positive cells were sorted using FACS Aria, and RNA was isolated from each population without cell expansion ( Supplementary Fig. 1d ). Reverse transcription polymerase chain reaction (RT–PCR) analysis demonstrated that the Venus gene was only expressed in Venus-positive cells ( Supplementary Fig. 1e ). We purified 2.0 μg total RNA from Venus-negative cells and 1.75 μg total RNA from Venus-positive cells and subjected it to microarray analysis using an Affymetrix Mouse Genome 430 2.0 Array. High chondrocyte gene expression was observed in Venus-positive cells by quantitative RT–PCR (RT–qPCR; Fig. 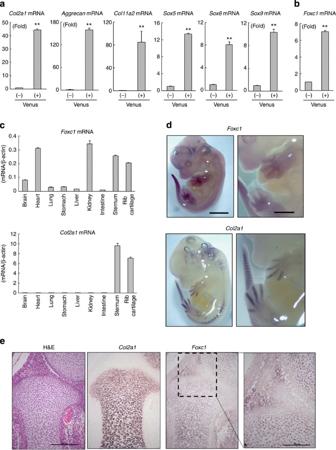Figure 1: Identification of Foxc1 as a candidate transcription factor selectively expressed in chondrocytes. (a,b) Total RNA isolated from Venus-negative and -positive cells was analysed by RT–qPCR for chondrocyte marker genes (a) andFoxc1(b) expression. Data are shown as the mean±s.d. (n=3). **P<0.01 (versus Venus (−)); Student’st-test. (c) Tissue distribution ofFoxc1(upper panel) andCol2a1(lower panel) mRNA in newborn mouse tissues. Total RNA isolated from indicated tissues was analysed by RT–qPCR. Data are shown as the mean±s.d. (n=3). (d) The expression ofFoxc1andCol2a1in developing limbs of E12.5 mice was determined by whole-mountin situhybridization. Scale bar, 2 mm (left panel), 1 mm (right panel). (e) Haematoxylin and eosin (H&E) staining andin situhybridization analysis ofCol2a1(middle panel) andFoxc1(right panel) in growth plate chondrocytes of E15.5 mice tibia. The boxed area shows higher magnification of distal chondrocytes. Scale bar, 200 μm (lower magnification, × 20) and 100 μm (higher magnification, × 40). 1a ) and microarray analysis ( Supplementary Table 1 ), indicating that purification of chondrocytes and gene expression profiling was successful. Microarray analysis, focusing on transcription factors, also showed that Sox5, Sox6 and Sox9 were highly expressed in Venus-positive cells ( Table 1 ). From the 10 most highly expressed transcription factors shown in Table 1 , we selected Foxc1 as a suitable candidate because human FOXC1 mutations cause the Axenfeld–Rieger syndrome, which is characterized by skeletal abnormalities [26] , [27] . However, the role of Foxc1 in chondrogenesis is unknown. Venus-positive cells expressed a high level of Foxc1, (1284) similar to that for Sox9 (1601; Table 1 ) and Foxc1 expression was increased by 7.03-fold compared with Venus-negative cells ( Fig. 1b ). Figure 1: Identification of Foxc1 as a candidate transcription factor selectively expressed in chondrocytes. ( a , b ) Total RNA isolated from Venus-negative and -positive cells was analysed by RT–qPCR for chondrocyte marker genes ( a ) and Foxc1 ( b ) expression. Data are shown as the mean±s.d. ( n =3). ** P <0.01 (versus Venus (−)); Student’s t -test. ( c ) Tissue distribution of Foxc1 (upper panel) and Col2a1 (lower panel) mRNA in newborn mouse tissues. Total RNA isolated from indicated tissues was analysed by RT–qPCR. Data are shown as the mean±s.d. ( n =3). ( d ) The expression of Foxc1 and Col2a1 in developing limbs of E12.5 mice was determined by whole-mount in situ hybridization. Scale bar, 2 mm (left panel), 1 mm (right panel). ( e ) Haematoxylin and eosin (H&E) staining and in situ hybridization analysis of Col2a1 (middle panel) and Foxc1 (right panel) in growth plate chondrocytes of E15.5 mice tibia. The boxed area shows higher magnification of distal chondrocytes. Scale bar, 200 μm (lower magnification, × 20) and 100 μm (higher magnification, × 40). Full size image Table 1 Ten most highly expressed transcription factors in Venus-positive cells. Full size table Expression of Foxc1 in chondrocytes We next used RT–qPCR to demonstrate high levels of Foxc1 expression in the sternum and rib cartilage, where Col2a1 is also highly expressed ( Fig. 1c ). Whole-mount in situ hybridization analysis of E12.5 mice revealed high Foxc1 expression in developing limb buds ( Fig. 1d ) and in situ hybridization analysis of E15.5 mouse tibias showed strong expression of Foxc1 in Col2a1 -positive chondrocytes ( Fig. 1e ). Importantly, Foxc1 mRNA was detected in distal chondrocytes, which are known to produce PTHrP ( Fig. 1e ). Immunohistochemical analysis of E13.5 developing limb buds also demonstrated that Foxc1 was detected not only in proliferating chondrocytes but also in perichondrial cells at the end of growth plates where PTHrP is synthesized ( Supplementary Fig. 2a ). Moreover, Foxc1 was expressed in resting, proliferating and hypertrophic chondrocytes in the tibial growth plates of newborn mice ( Supplementary Fig. 2b ). These data collectively suggest that Foxc1 might play multifunctional roles during both early and late endochondral ossification. Foxc1 is critical for endochondral ossification in vivo Using a spontaneous loss of Foxc1 function mutant mouse ( Foxc1 ch/ch ), we determined the in vivo significance of Foxc1 during endochondral ossification. Foxc1 ch/ch mice died soon after birth and showed abnormal skeletal development, as previously described [28] . Skeletal preparations of newborn Foxc1 ch/ch mice showed a reduction in Alcian Blue staining, no ossification centre in the sternum and impaired calcification in vertebrae compared with wild-type (WT) mice ( Supplementary Fig. 3a,b ). Moreover, Foxc1 ch/ch mice exhibited significantly shorter limbs than WT ( Supplementary Fig. 3c–e ). Consistent with this, histological analysis of femurs ( Fig. 2a ) and tibias ( Supplementary Fig. 3f ) of newborn mice also showed weaker Alcian Blue staining and a smaller ossification centre in Foxc1 ch/ch mice compared with WT littermates. Notably, the sternum phenotype was characterized by disorganized rib fusion, the complete absence of hypertrophic chondrocytes and ossification ( Fig. 2b ). Further analysis of tibial growth plate chondrocytes revealed that the Foxc1 ch/ch hypertrophic chondrocyte zone was significantly longer than that of WT mice ( Fig. 2c,d ). These data suggest that Foxc1 inactivation disrupts endochondral ossification, leading to an abnormal skeletal phenotype. 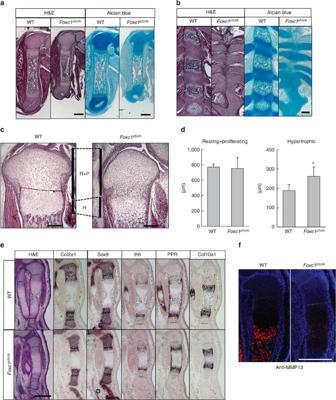Figure 2: Delayed endochondral ossification inFoxc1ch/chmice. (a,b) Histological analysis of newborn WT andFoxc1ch/chlittermate femurs (a) and sternums (b). Paraffin sections of femurs and sternums from newborn WT andFoxc1ch/chlittermates were examined by haematoxylin and eosin (H&E) and Alcian blue staining. Scale bar, (a) 500 μm. (b) 200 μm. (c) Histological analysis of tibial growth plate chondrocytes of newborn WT andFoxc1ch/chlittermates. H, hypertrophic chondrocytes; P, proliferating chondrocytes; R, resting chondrocytes. Scale bar 200 μm. (d) Quantitative analysis of the lengths of the resting and proliferating zone (Resting+Proliferating) and the hypertrophic zone (Hypertrophic) was performed using H&E-stained sections of the tibia. Data are shown as the mean±s.d. (n=6). *P<0.05 (versus WT); Student’st-test. (e) Paraffin sections of tibia from E15.5 WT andFoxc1ch/chlittermate embryos were examined by H&E staining andin situhybridization using antisense probes againstCol2a1,Sox9,Ihh,PPRandCol10a1. Scale bar, 500 μm. (f) Paraffin sections of tibia from E15.5 WT andFoxc1ch/chlittermates were subjected to immunofluorescence analyses using an anti-MMP13 antibody. Scale bar, 500 μm. Figure 2: Delayed endochondral ossification in Foxc1 ch/ch mice. ( a , b ) Histological analysis of newborn WT and Foxc1 ch/ch littermate femurs ( a ) and sternums ( b ). Paraffin sections of femurs and sternums from newborn WT and Foxc1 ch/ch littermates were examined by haematoxylin and eosin (H&E) and Alcian blue staining. Scale bar, ( a ) 500 μm. ( b ) 200 μm. ( c ) Histological analysis of tibial growth plate chondrocytes of newborn WT and Foxc1 ch/ch littermates. H, hypertrophic chondrocytes; P, proliferating chondrocytes; R, resting chondrocytes. Scale bar 200 μm. ( d ) Quantitative analysis of the lengths of the resting and proliferating zone (Resting+Proliferating) and the hypertrophic zone (Hypertrophic) was performed using H&E-stained sections of the tibia. Data are shown as the mean±s.d. ( n =6). * P <0.05 (versus WT); Student’s t -test. ( e ) Paraffin sections of tibia from E15.5 WT and Foxc1 ch/ch littermate embryos were examined by H&E staining and in situ hybridization using antisense probes against Col2a1 , Sox9 , Ihh , PPR and Col10a1 . Scale bar, 500 μm. ( f ) Paraffin sections of tibia from E15.5 WT and Foxc1 ch/ch littermates were subjected to immunofluorescence analyses using an anti-MMP13 antibody. Scale bar, 500 μm. Full size image To further investigate endochondral ossification in Foxc1 ch/ch mice, we investigated embryonic growth plate chondrocytes. Foxc1 ch/ch mice at E15.5 showed a slight dwarf phenotype and smaller ossification areas ( Supplementary Fig. 4a,b ), and haematoxylin and eosin (H&E) staining of E15.5 tibias demonstrated degradation of the hypertrophic chondrocyte zone in the centre of WT but not Foxc1 ch/ch tibias ( Fig. 2e ). In situ hybridization analysis of E15.5 tibias revealed a reduced and delayed Col10a1 -positive zone in Foxc1 ch/ch mice compared with that of WT mice, whereas the expression patterns of other chondrocyte genes were unchanged ( Fig. 2e ). Immunofluorescence analysis also showed a decrease in the Col10-positive area and a delay of Col10 expression in Foxc1 ch/ch mice compared with that in WT mice ( Supplementary Fig. 4c ). Moreover, MMP13 expression was markedly diminished ( Fig. 2f ) and the invasion of Col1a1 - and Runx2 -positive osteoblasts was not observed in Foxc1 ch/ch mice ( Supplementary Fig. 4d ), suggesting retarded chondrocyte hypertrophy. Collectively, these data suggest that Foxc1 ch/ch mice exhibit abnormal skeletal development because of a delay in endochondral ossification. Foxc1 directly regulates PTHrP expression We next examined the functional role of Foxc1 in endochondral ossification. Because Foxc1 protein is expressed in resting, proliferating and hypertrophic chondrocytes ( Supplementary Fig. 2b ), we reasoned that it must be involved in both early and late stages of endochondral ossification. This idea is consistent with results observed in Foxc1 ch/ch mice ( Fig. 2a–c , Supplementary Fig. 3 ). To test this, we used RT–qPCR to identify Foxc1 target genes in resting and proliferating chondrocytes. When Foxc1 was overexpressed in primary chondrocytes, it markedly increased PTHrP expression ( Fig. 3a ). Together with our earlier immunohistochemical analysis ( Supplementary Fig. 2a ), which showed the expression of Foxc1 in perichondrial cells at the end of growth plates, this suggests that PTHrP is a target gene of Foxc1 in the early stage of chondrocyte development. In support of this, the PTHrP promoter was found to contain a motif that fits the core consensus Foxc1-binding sequence [29] ( Fig. 3b ). DNA pull-down assays using the biotinylated Foxc1-binding element demonstrated that Foxc1 directly bound to this element and that binding was markedly competed with by excess non-biotinylated probe in a dose-dependent manner ( Fig. 3b ). Chromatin immunoprecipitation (ChIP) with an anti-Foxc1 antibody showed the direct binding of Foxc1 to the PTHrP promoter ( Fig. 3c ). Moreover, Foxc1 increased the promoter activity of a reporter construct containing six copies of the Foxc1-binding element from the PTHrP promoter in a dose-dependent manner ( Fig. 3d ). Foxc1 was further shown to regulate PTHrP expression because mRNA isolated from Foxc1 ch/ch limbs had reduced levels of PTHrP mRNA compared with that from WT limbs ( Fig. 3e ). Of note, a BrdU labelling assay demonstrated that Foxc1 ch/ch chondrocytes had a significantly decreased proliferation rate compared with that of WT chondrocytes, suggesting that the Foxc1-dependent PTHrP action in growth plate chondrocytes was impaired in Foxc1 ch/ch mice ( Supplementary Fig. 5 ). Taken together, these data indicate that PTHrP is likely to be a direct target gene of Foxc1 in chondrocytes. 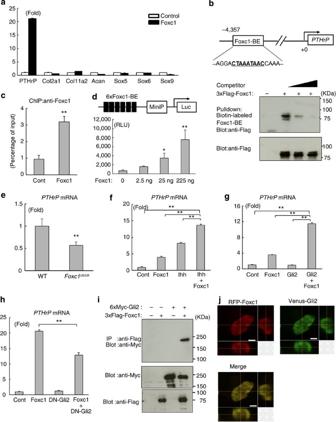Figure 3: Foxc1 regulatesPTHrPexpression through physical and functional interaction with Ihh–Gli2 signalling. (a) Effects of Foxc1 on chondrocyte gene expression in primary chondrocytes analysed by RT–qPCR. (b) DNA pull-down assays using the Foxc1-binding element in thePTHrPgene promoter. Schematic presentation of the putative Foxc1-binding element (CTAAATAAC) in the mousePTHrPgene promoter (top panel). 293FT cell lysates precipitated with biotin-labelled Foxc1-BE oligonucleotide (middle panel) and cell lysates (bottom panel) were determined by immunoblotting with an anti-Flag antibody. (c)Foxc1was overexpressed in primary chondrocytes and ChIP assays were performed using anti-Foxc1 antibody. The binding of Foxc1 to thePTHrPgene promoter was examined by qPCR. **P<0.01 (versus Control); Student’st-test. (d) COS-7 cells were transfected with reporter constructs containing 6xFoxc1-BE from thePTHrPgene promoter (upper panel) together with an empty vector and Foxc1. RLU, relative luciferase units. *P<0.05, **P<0.01(versus 0 ng) (e)PTHrPmRNA expression was determined by RT–qPCR using microdissected hindlimbs isolated from E15.5Foxc1ch/chand WT littermate fetuses **P<0.01 (versus WT); Student’st-test. (f,g) Synergistic effect of Foxc1 and Ihh (f) and Foxc1 and Gli2 (g) onPTHrPmRNA expression in primary chondrocytes 3 days after infection with the indicated adenoviruses. **P<0.01 (versus Control, Foxc1 or Ihh) **P<0.01 (versus Control, Foxc1 or Gli2). (h) Effect of DN-Gli2 on Foxc1-dependentPTHrPmRNA expression in primary chondrocytes 6 days after infection with the indicated adenoviruses; **P<0.01 (versus Foxc1). Data for (a,c,d–h) are shown as mean±s.d. (n=3) and statistical analysis (d,f,g,h) was performed by one-way analysis of variance followed by the Tukey–Kramer test. (i) 293FT cell lysates were immunoprecipitated with an anti-Flag antibody and then immunoblotted with an anti-Myc antibody (top panel). The cell lysates were immunoblotted with an anti-Myc (middle panel) or anti-Flag (bottom panel) antibody. (j) HEK293 cells were transfected with both RFP-tagged-Foxc1 (RFP-Foxc1) and Venus-tagged Gli2 (Venus-Gli2). Confocal cross sections ofxy(left),yz(right) andxz(bottom) were visualized under a confocal microscope. Scale bar, 5 μm. Figure 3: Foxc1 regulates PTHrP expression through physical and functional interaction with Ihh–Gli2 signalling. ( a ) Effects of Foxc1 on chondrocyte gene expression in primary chondrocytes analysed by RT–qPCR. ( b ) DNA pull-down assays using the Foxc1-binding element in the PTHrP gene promoter. Schematic presentation of the putative Foxc1-binding element (CTAAATAAC) in the mouse PTHrP gene promoter (top panel). 293FT cell lysates precipitated with biotin-labelled Foxc1-BE oligonucleotide (middle panel) and cell lysates (bottom panel) were determined by immunoblotting with an anti-Flag antibody. ( c ) Foxc1 was overexpressed in primary chondrocytes and ChIP assays were performed using anti-Foxc1 antibody. The binding of Foxc1 to the PTHrP gene promoter was examined by qPCR. ** P <0.01 (versus Control); Student’s t -test. ( d ) COS-7 cells were transfected with reporter constructs containing 6xFoxc1-BE from the PTHrP gene promoter (upper panel) together with an empty vector and Foxc1. RLU, relative luciferase units. * P <0.05, ** P <0.01(versus 0 ng) ( e ) PTHrP mRNA expression was determined by RT–qPCR using microdissected hindlimbs isolated from E15.5 Foxc1 ch/ch and WT littermate fetuses ** P <0.01 (versus WT); Student’s t -test. ( f , g ) Synergistic effect of Foxc1 and Ihh ( f ) and Foxc1 and Gli2 ( g ) on PTHrP mRNA expression in primary chondrocytes 3 days after infection with the indicated adenoviruses. ** P <0.01 (versus Control, Foxc1 or Ihh) ** P <0.01 (versus Control, Foxc1 or Gli2). ( h ) Effect of DN-Gli2 on Foxc1-dependent PTHrP mRNA expression in primary chondrocytes 6 days after infection with the indicated adenoviruses; ** P <0.01 (versus Foxc1). Data for ( a , c , d – h ) are shown as mean±s.d. ( n =3) and statistical analysis ( d , f , g , h ) was performed by one-way analysis of variance followed by the Tukey–Kramer test. ( i ) 293FT cell lysates were immunoprecipitated with an anti-Flag antibody and then immunoblotted with an anti-Myc antibody (top panel). The cell lysates were immunoblotted with an anti-Myc (middle panel) or anti-Flag (bottom panel) antibody. ( j ) HEK293 cells were transfected with both RFP-tagged-Foxc1 (RFP-Foxc1) and Venus-tagged Gli2 (Venus-Gli2). Confocal cross sections of xy (left), yz (right) and xz (bottom) were visualized under a confocal microscope. Scale bar, 5 μm. Full size image Foxc1 regulates Ihh target gene expression with Gli2 Accumulating evidence shows that Ihh and its major signalling molecule, Gli2, regulate PTHrP expression in chondrocytes [15] , [30] . For example, the targeted disruption of Gli2 in mice causes a reduction in PTHrP expression and abnormal endochondral ossification [17] . These reports led us to hypothesize that Foxc1 associates with Ihh–Gli2 signalling in the regulation of PTHrP . We observed no significant difference in Ihh mRNA levels between Foxc1 ch/ch and WT mice ( Supplementary Fig. 6a ). In addition, the overexpression of Foxc1 had no effect on Ihh mRNA levels in the presence or absence of Gli2 ( Supplementary Fig. 6b ). These data suggest that Foxc1 does not affect Ihh expression. In contrast, the concomitant expression of Foxc1 and Ihh in primary chondrocytes increased PTHrP expression to levels higher than that induced by Ihh alone ( Fig. 3f ). These data suggest a functional cooperation between Foxc1 and intracellular signalling activated by Ihh. Notably, a synergistic effect between Foxc1 and Gli2 was observed to affect PTHrP expression in primary chondrocytes ( Fig. 3g ), while a dominant negative (DN) Gli2 decreased Foxc1-dependent PTHrP expression ( Fig. 3h ). Moreover, immunoprecipitation (IP)-western analysis revealed that Foxc1 physically associates with Gli2 ( Fig. 3i ). In addition, red fluorescent protein (RFP)-tagged Foxc1 co-localized with Venus-tagged Gli2 in the nucleus ( Fig. 3j ). Collectively, these data suggest that Foxc1 regulates PTHrP expression through its functional and physical interaction with Ihh–Gli2 signalling. In addition to PTHrP , Ihh–Gli2 signalling also directly controls the expression of several genes during endochondral ossification, including Gli1 and Ptch1 (ref. 12 ). Thus, we next determined whether Foxc1, with the involvement of Ihh–Gli2 signalling, modulates Gli1 and Ptch1 expression. Although Foxc1 alone failed to increase Gli1 and Ptch1 mRNA levels in primary chondrocytes, it could stimulate Gli1 and Ptch1 expression induced by Ihh ( Fig. 4a,b ). Consistent with the PTHrP mRNA induction ( Fig. 3g ), the concomitant overexpression of Foxc1 and Gli2 synergistically increased Gli1 and Ptch1 expression levels in primary chondrocytes ( Fig. 4c,d ). It should be noted that Gli1 and Ptch1 expression in Foxc1 ch/ch tibias was reduced compared with that in WT mice ( Fig. 4e,f ). Moreover, Foxc1 increased the binding of Gli2 to the Gli-binding element located in the PTHrP , Gli1 (ref. 31 ) and Ptch1 (ref. 32 ) promoters, as shown by ChIP assays using an anti-Gli2 antibody ( Fig. 4g–i ). Of note, the binding activity of endogenous Gli2 to the Gli-binding element located in the PTHrP , Gli1 and Ptch1 gene promoters was significantly decreased in Foxc1 ch/ch chondrocytes compared with that in WT chondrocytes ( Supplementary Fig. 7 ). These results collectively suggest that Foxc1, as a transcriptional partner of Gli2, promotes the expression of Ihh target genes, which, in turn, regulates endochondral ossification. 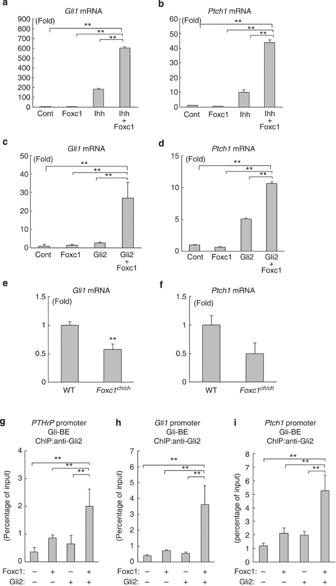Figure 4: Foxc1 controls the expression of Ihh target genes by recruiting Gli2. (a,b) Synergistic effect of Foxc1 and Ihh onGli1(a) andPtch1(b) mRNA expression in primary chondrocytes infected with adenoviruses as indicated. Data are shown as the mean±s.d. (n=3). **P<0.01 (versus Control, Foxc1 or Ihh); one-way analysis of variance (ANOVA) followed by the Tukey–Kramer test. (c,d) Synergistic effect of Foxc1 and Gli2 onGli1(c) andPtch1(d) mRNA expression in primary chondrocytes infected with adenoviruses as indicated. Data are shown as the mean±s.d. (n=3). **P<0.01 (versus Control, Foxc1 or Gli2); one-way ANOVA followed by the Tukey–Kramer test. (e,f) Total RNA was isolated from the microdissected hindlimbs of E15.5 WT andFoxc1ch/chlittermate embryos, andGli1(e) andPtch1(f) mRNA expression was determined by RT–qPCR. Data are shown as fold expression normalized to WT (mean±s.d.,n=3). **P<0.01 (versus WT); Student’st-test. (g–i) Primary chondrocytes were infected with control, Foxc1, Gli2 or both Foxc1 and Gli2 adenoviruses and cultured for 3 days. ChIP assays were conducted using an anti-Gli2 antibody and DNA binding to gene promoters was determined by qPCR using primer pairs specific forPTHrP(g),Gli1(h) andPtch1(i) gene promoters, which contain the Gli-binding element. Data are shown as the mean±s.d. (n=3). **P<0.01 (versus control, Foxc1, or Gli2); one-way ANOVA followed by the Tukey–Kramer test. Figure 4: Foxc1 controls the expression of Ihh target genes by recruiting Gli2. ( a , b ) Synergistic effect of Foxc1 and Ihh on Gli1 ( a ) and Ptch1 ( b ) mRNA expression in primary chondrocytes infected with adenoviruses as indicated. Data are shown as the mean±s.d. ( n =3). ** P <0.01 (versus Control, Foxc1 or Ihh); one-way analysis of variance (ANOVA) followed by the Tukey–Kramer test. ( c , d ) Synergistic effect of Foxc1 and Gli2 on Gli1 ( c ) and Ptch1 ( d ) mRNA expression in primary chondrocytes infected with adenoviruses as indicated. Data are shown as the mean±s.d. ( n =3). ** P <0.01 (versus Control, Foxc1 or Gli2); one-way ANOVA followed by the Tukey–Kramer test. ( e , f ) Total RNA was isolated from the microdissected hindlimbs of E15.5 WT and Foxc1 ch/ch littermate embryos, and Gli1 ( e ) and Ptch1 ( f ) mRNA expression was determined by RT–qPCR. Data are shown as fold expression normalized to WT (mean±s.d., n =3). ** P <0.01 (versus WT); Student’s t -test. ( g – i ) Primary chondrocytes were infected with control, Foxc1, Gli2 or both Foxc1 and Gli2 adenoviruses and cultured for 3 days. ChIP assays were conducted using an anti-Gli2 antibody and DNA binding to gene promoters was determined by qPCR using primer pairs specific for PTHrP ( g ), Gli1 ( h ) and Ptch1 ( i ) gene promoters, which contain the Gli-binding element. Data are shown as the mean±s.d. ( n =3). ** P <0.01 (versus control, Foxc1, or Gli2); one-way ANOVA followed by the Tukey–Kramer test. Full size image Col10a1 is a target gene of Foxc1 in chondrocytes Foxc1 is expressed in hypertrophic chondrocytes ( Supplementary Fig. 2b ); therefore, we next examined its role in the late stage of endochondral ossification. We overexpressed Foxc1 in primary chondrocytes and evaluated the expression of hypertrophic chondrocyte marker genes. Foxc1 markedly upregulated Col10a1 expression ( Fig. 5a ). The Col10a1 promoter has a putative Foxc1-binding motif in the opposite orientation to that of Col10a1 transcription ( Fig. 5b ). DNA pull-down assays using a biotinylated form of this Foxc1-binding element demonstrated the direct binding of Foxc1, which could be competed with by an excess of non-biotinylated probe ( Fig. 5c ). ChIP assays using an anti-Foxc1 antibody also revealed that Foxc1 bound to the Col10a1 promoter ( Fig. 5d ). Moreover, Foxc1 increased the promoter activity of a reporter construct containing six copies of the Col10a1 promoter Foxc1-binding element ( Fig. 5e ), similar to the experiment in Fig. 3d . Taken together, these results suggest that Col10a1 is a direct target gene of Foxc1 during the late stage of endochondral ossification. 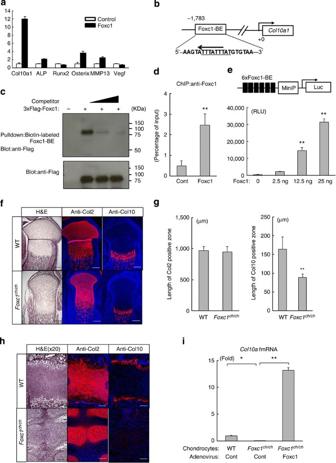Figure 5: Col10a1 is the direct target of Foxc1in vitroandin vivo. (a) Effects of Foxc1 on hypertrophic chondrocyte gene expression. Primary chondrocytes were infected with control or Foxc1 adenovirus and chondrocyte gene expression was analysed by RT–qPCR. Data are shown as the mean±s.d. (n=3). (b) Schematic presentation of the putative Foxc1-binding element (ATTTATTTA) in the promoter region of mouseCol10a1. (c) DNA pull-down assays using the Foxc1-binding element in theCol10a1promoter. 293FT cell lysates precipitated with biotin-labelled Foxc1-BE oligonucleotide (upper) and total cell lysates (lower) were assessed by immunoblotting with an anti-Flag antibody. (d) ChIP assays using anti-Foxc1 antibody. The binding of Foxc1 to theCol10a1promoter was examined by qPCR. Data are shown as the mean±s.d. (n=6). **P<0.01 (versus Control); Student’st-test. (e) COS-7 cells were transfected with reporter constructs containing 6xFoxc1-BE from theCol10a1gene promoter (upper panel) together with an empty vector and Foxc1. Data are expressed in relative luciferase units (mean±s.d.,n=3). **P<0.01 (versus 0 ng); one-way analysis of variance (ANOVA) followed by the Tukey–Kramer test. (f) Immunofluorescence analysis of tibial growth plate chondrocytes in newborn WT andFoxc1ch/chlittermates. Paraffin sections of tibia were subjected to haematoxylin and eosin (H&E) staining and immunofluorescence analyses using anti-Col2 and anti-Col10 antibodies. Scale bar, 200 μm. (g) Quantitative analysis of the lengths of Col2-positive and Col10-positive zones. Data are shown as the mean±s.d. (n=5) **P<0.01 (versus WT); Student’st-test. (h) Immunofluorescence analysis of sternums in newborn WT andFoxc1ch/chmice. Paraffin sections of sternums of the mice were subjected to immunofluorescence analyses using an anti-Col2 or anti-Col10 antibody. The H&E staining images are higher magnification images of those presented inFig. 2b. Scale bar, 100 μm. (i) Primary chondrocytes from E18.5 WT andFoxc1ch/chlittermates were infected with control (Cont) or Foxc1 adenovirus as indicated.Col10a1mRNA expression was determined by RT–qPCR. Data are shown as the mean±s.d. (n=3) **P<0.01, *P<0.05; one-way ANOVA followed by the Tukey–Kramer test. Figure 5: Col10a1 is the direct target of Foxc1 in vitro and in vivo . ( a ) Effects of Foxc1 on hypertrophic chondrocyte gene expression. Primary chondrocytes were infected with control or Foxc1 adenovirus and chondrocyte gene expression was analysed by RT–qPCR. Data are shown as the mean±s.d. ( n =3). ( b ) Schematic presentation of the putative Foxc1-binding element (ATTTATTTA) in the promoter region of mouse Col10a1 . ( c ) DNA pull-down assays using the Foxc1-binding element in the Col10a1 promoter. 293FT cell lysates precipitated with biotin-labelled Foxc1-BE oligonucleotide (upper) and total cell lysates (lower) were assessed by immunoblotting with an anti-Flag antibody. ( d ) ChIP assays using anti-Foxc1 antibody. The binding of Foxc1 to the Col10a1 promoter was examined by qPCR. Data are shown as the mean±s.d. ( n =6). ** P <0.01 (versus Control); Student’s t -test. ( e ) COS-7 cells were transfected with reporter constructs containing 6xFoxc1-BE from the Col10a1 gene promoter (upper panel) together with an empty vector and Foxc1. Data are expressed in relative luciferase units (mean±s.d., n =3). ** P <0.01 (versus 0 ng); one-way analysis of variance (ANOVA) followed by the Tukey–Kramer test. ( f ) Immunofluorescence analysis of tibial growth plate chondrocytes in newborn WT and Foxc1 ch/ch littermates. Paraffin sections of tibia were subjected to haematoxylin and eosin (H&E) staining and immunofluorescence analyses using anti-Col2 and anti-Col10 antibodies. Scale bar, 200 μm. ( g ) Quantitative analysis of the lengths of Col2-positive and Col10-positive zones. Data are shown as the mean±s.d. ( n =5) ** P <0.01 (versus WT); Student’s t -test. ( h ) Immunofluorescence analysis of sternums in newborn WT and Foxc1 ch/ch mice. Paraffin sections of sternums of the mice were subjected to immunofluorescence analyses using an anti-Col2 or anti-Col10 antibody. The H&E staining images are higher magnification images of those presented in Fig. 2b . Scale bar, 100 μm. ( i ) Primary chondrocytes from E18.5 WT and Foxc1 ch/ch littermates were infected with control (Cont) or Foxc1 adenovirus as indicated. Col10a1 mRNA expression was determined by RT–qPCR. Data are shown as the mean±s.d. ( n =3) ** P <0.01, * P <0.05; one-way ANOVA followed by the Tukey–Kramer test. Full size image To determine whether Foxc1 regulates Col10a1 expression during endochondral ossification in vivo , we carried out immunofluorescence analysis of tibial growth plates from newborn mice. This revealed that the type-10 collagen-positive zone was significantly shorter in Foxc1 ch/ch compared with WT mice, while the type-2 collagen-positive zone was unchanged ( Fig. 5f,g ). In addition, impaired Col10 expression in growth plate chondrocytes was also observed in E15.5 and E17.5 tibia of Foxc1 ch/ch mice ( Supplementary Figs 4c and 8). Analysis of the newborn sternum demonstrated that type-2 collagen-positive chondrocytes failed to undergo sternum development and that type-10 collagen-positive chondrocytes were not detected in Foxc1 ch/ch mice ( Fig. 5h ), suggesting impaired chondrocyte hypertrophy. RT–qPCR analysis using primary chondrocytes revealed that Col10a1 mRNA levels were strikingly decreased in Foxc1 ch/ch compared with WT mice ( Fig. 5i ). Importantly, the decrease of Col10a1 expression in Foxc1 ch/ch mice was restored by the overexpression of Foxc1 ( Fig. 5i ). Collectively, these results showed that Foxc1-dependent regulation of Col10a1 expression is important for endochondral ossification. DN-Foxc1 reduced Ihh target gene expression To gain further insight into the role of Foxc1 in chondrogenesis, we examined the effect of a Foxc1 mutant on Ihh target gene expression. We generated a DN mutant of Foxc1 (DN-Foxc1) containing a DNA-binding domain and a transcriptional inhibitory domain [33] ( Supplementary Fig. 9a,b ). DN-Foxc1 inhibited the transcriptional activity of WT Foxc1 as assessed by a reporter assay ( Supplementary Fig. 9c ). Overexpression of DN-Foxc1 decreased PTHrP and Col10a1 expression induced by Foxc1 in primary chondrocytes ( Supplementary Fig. 9d,e ). Of note, DN-Foxc1 also decreased the expression of PTHrP , Gli1 , Ptch1 and Col10a1 induced by Ihh ( Supplementary Fig. 9f–i ). These results indicate the importance of Foxc1 in the chondrogenic action of Ihh. Functional redundancy between Foxc1 and Foxc2 Although we have shown that Foxc1 controls PTHrP expression, which is essential for endochondral ossification, the skeletal phenotype of Foxc1 ch/ch long bones was relatively mild compared with the severe skeletal defects previously observed in PTHrP-deficient mice [34] , [35] . Of the forkhead transcription factor superfamily [36] , Foxc2 is the most closely related to Foxc1 and Nifuji et al reported the expression of Foxc2 in perichondrium [37] . Thus, we reasoned that the mild skeletal defect observed in Foxc1 ch/ch mice was likely caused by the functional redundancy between Foxc1 and Foxc2. To support this notion, our microarray analysis and RT–qPCR analysis revealed high levels of Foxc2 expression in chondrogenic cells ( Table 1 and Supplementary Fig. 10a ). Foxc2 was also relatively highly expressed in the cartilage tissues of newborn mice ( Supplementary Fig. 10b ), while immunohistochemical analysis using an anti-Foxc2 antibody revealed Foxc2 expression in resting, proliferating and hypertrophic chondrocytes of the tibial growth plate ( Supplementary Fig. 10c ). Interestingly, Foxc2 increased PTHrP and Col10a1 expression in primary chondrocytes and stimulated reporter activity through either PTHrP or Col10a1 promoter Foxc1-binding elements ( Supplementary Fig. 10d–g ). However, the synergistic effects of Foxc2 and Gli2 on Ihh target gene expression, including for PTHrP , Gli1 and Ptch1 , were significant but very weak ( Supplementary Fig. 10h–j ) compared with those of Foxc1 ( Figs 3g and 4c,d ). We next compared the expression level of Foxc1 and Foxc2 in chondrocytes. We found stronger expression of Foxc1 in growth plate chondrocytes compared with that of Foxc2 as determined by in situ hybridization analysis ( Supplementary Fig. 11a ). RT–PCR analysis also showed a low level of Foxc2 mRNA in rib cartilage and primary chondrocytes, while the level of Foxc2 mRNA was approximately equivalent to that of Foxc1 mRNA in kidney ( Supplementary Fig. 11b ). Taken together, these data suggest that Foxc2 has a similar function but does not completely overlap with that of Foxc1 in endochondral ossification. A Foxc1 missense mutation failed to interact with Gli2 The Axenfeld–Rieger syndrome, characterized by glaucoma, hypodontia and skeletal abnormalities, including facial dysmorphism and short stature, is caused by mutations in FOXC1 (refs 27 , 38 , 39 ). Interestingly, mutations of PTHLH , a human homologue of PTHrP , cause brachydactyly and a similar disorder in which patients have a short stature and missing teeth [40] . These clinical observations suggest clinical relevance for the Foxc1–PTHrP axis in the Axenfeld–Rieger syndrome. Thus, we next investigated the pathological role of the FOXC1 mutation, Phe112Ser (F112S), previously identified in the Axenfeld–Rieger syndrome [26] , [41] . We confirmed that the expression of the mutant protein F112S was equivalent to that of WT Foxc1 ( Fig. 6a ). Transfection of the F112S mutant decreased PTHrP expression and transcriptional activity of Foxc1, suggesting that F112S acts in a dominant negative manner ( Fig. 6b,c ). F112S also decreased Ihh-dependent PTHrP expression ( Fig. 6d ). Moreover, the functional interaction between Foxc1 and Gli2 was strikingly attenuated in the F112S transfectant, which, in turn, impaired PTHrP induction ( Fig. 6e ). Although F112S could bind the Foxc1-binding element in the PTHrP promoter ( Fig. 6f ), IP-western analysis demonstrated that F112S failed to physically interact with Gli2 ( Fig. 6g ). RFP-tagged-Foxc1-F112S localized to the nucleus but showed an abnormal aggregation pattern, which resulted in a marked reduction of nuclear co-localization with Venus-tagged Gli2 ( Fig. 6h ). Furthermore, F112S failed to recruit endogenous Gli2 to the Gli-binding element located in the PTHrP , Gli1 and Ptch1 gene promoters ( Supplementary Fig. 12 ). These results collectively suggest that the loss of functional interaction between F112S and Gli2 contribute, at least in part, to the pathogenesis of the Axenfeld–Rieger syndrome. 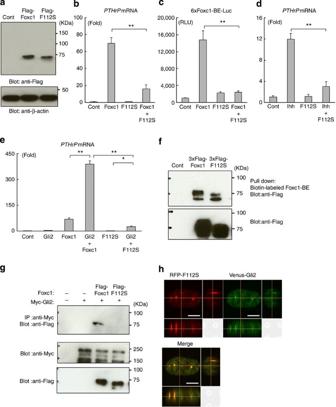Figure 6: Impaired functional interaction between a pathological missenseFoxc1mutant and Gli2. (a) 293FT cells were transfected with empty vector, Flag-tagged WT Foxc1 (Flag–Foxc1) or Flag-tagged-F112S mutant Foxc1 (Flag-F112S), and cell lysates were immunoblotted with anti-Flag (upper panel) and anti-β-actin (lower panel) antibodies. (b) Effect of F112S mutant on PTHrP.PTHrPmRNA expression was determined by RT–qPCR. Data are shown as fold activation normalized to control (mean±s.d.,n=3). **P<0.01 (versus Foxc1); one-way analysis of variance (ANOVA) followed by the Tukey–Kramer test. (c) Effect of the F112S mutation on Foxc1 transcriptional activity on thePTHrPpromoter. Data are expressed in relative luciferase units (mean±s.d.,n=3). **P<0.01 (versus Foxc1); one-way ANOVA followed by the Tukey–Kramer test. (d) Inhibitory effect of F112S onPTHrPmRNA expression induced by Ihh. Data are shown as the mean±s.d. (n=3). **P<0.01(versus Ihh); one-way ANOVA followed by the Tukey–Kramer test. (e) Impaired synergistic effect between F112S and Gli2 onPTHrPmRNA expression. Primary chondrocytes were infected with the indicated adenoviruses andPTHrPmRNA expression was analysed by RT–qPCR analysis. Data are shown as the mean±s.d. (n=3). **P<0.01, *P<0.05; one-way ANOVA followed by the Tukey–Kramer test. (f) DNA pull-down assays using the Foxc1-binding element from thePTHrPpromoter. Samples precipitated with the biotin-labelled Foxc1-BE oligonucleotide (upper panel) and total cell lysates (lower panel) were immunoblotted with an anti-Flag antibody. (g) F112S failed to interact with Gli2. Lysates of the 293FT cells transfected as indicated were immunoprecipitated with an anti-Myc antibody and immunoblotted with an anti-Flag antibody (top). The cell lysates were immunoblotted with an anti-Myc (middle) or anti-Flag (bottom) antibody. (h) Nuclear localization of F112S and Gli2. HEK293 cells transfected with RFP-tagged F112S (RFP-F112S) and Venus-tagged Gli2 (Venus-Gli2). Confocal cross sections ofxy(top left),yz(right) andxz(bottom) were visualized under a confocal microscope. Scale bar, 5 μm. Figure 6: Impaired functional interaction between a pathological missense Foxc1 mutant and Gli2. ( a ) 293FT cells were transfected with empty vector, Flag-tagged WT Foxc1 (Flag–Foxc1) or Flag-tagged-F112S mutant Foxc1 (Flag-F112S), and cell lysates were immunoblotted with anti-Flag (upper panel) and anti-β-actin (lower panel) antibodies. ( b ) Effect of F112S mutant on PTHrP. PTHrP mRNA expression was determined by RT–qPCR. Data are shown as fold activation normalized to control (mean±s.d., n =3). ** P <0.01 (versus Foxc1); one-way analysis of variance (ANOVA) followed by the Tukey–Kramer test. ( c ) Effect of the F112S mutation on Foxc1 transcriptional activity on the PTHrP promoter. Data are expressed in relative luciferase units (mean±s.d., n =3). ** P <0.01 (versus Foxc1); one-way ANOVA followed by the Tukey–Kramer test. ( d ) Inhibitory effect of F112S on PTHrP mRNA expression induced by Ihh. Data are shown as the mean±s.d. ( n =3). ** P <0.01(versus Ihh); one-way ANOVA followed by the Tukey–Kramer test. ( e ) Impaired synergistic effect between F112S and Gli2 on PTHrP mRNA expression. Primary chondrocytes were infected with the indicated adenoviruses and PTHrP mRNA expression was analysed by RT–qPCR analysis. Data are shown as the mean±s.d. ( n =3). ** P <0.01, * P <0.05; one-way ANOVA followed by the Tukey–Kramer test. ( f ) DNA pull-down assays using the Foxc1-binding element from the PTHrP promoter. Samples precipitated with the biotin-labelled Foxc1-BE oligonucleotide (upper panel) and total cell lysates (lower panel) were immunoblotted with an anti-Flag antibody. ( g ) F112S failed to interact with Gli2. Lysates of the 293FT cells transfected as indicated were immunoprecipitated with an anti-Myc antibody and immunoblotted with an anti-Flag antibody (top). The cell lysates were immunoblotted with an anti-Myc (middle) or anti-Flag (bottom) antibody. ( h ) Nuclear localization of F112S and Gli2. HEK293 cells transfected with RFP-tagged F112S (RFP-F112S) and Venus-tagged Gli2 (Venus-Gli2). Confocal cross sections of xy (top left), yz (right) and xz (bottom) were visualized under a confocal microscope. Scale bar, 5 μm. Full size image Endochondral ossification is characterized by sequential chondrocyte differentiation including resting, proliferating and hypertrophic processes. Chondrocytes form growth plate layers in which specific marker gene expression is strictly controlled by the communication of various transcription factors. Many details of this transcriptional network remain to be elucidated and to achieve a full understanding of the molecular basis of endochondral ossification it is important to identify and characterize the full repertoire of transcription factors involved. In this study, we performed FACS-assisted microarray profiling using transgenic mouse embryos that selectively express the Venus gene in developing chondrocytes. We identified Foxc1 as a functional transcription factor selectively expressed in chondrocytes under physiological conditions. Foxc1 has a diverse range of biological functions and is essential for the development of several tissues including the heart, blood vessels [42] , kidney and urinary tract [43] , the eye [44] and bones [45] . The mechanism by which Foxc1 regulates skeletal development has previously been investigated from the viewpoint of intramembranous bone formation with particular focus on osteoblasts, not endochondral ossification. Thus, several groups have reported the importance of bone morphogenetic protein signalling and Msx2 in Foxc1-dependent calvarial bone development [46] , [47] , [48] . Although Alcian blue-positive nodule formation of mesenchymal cells isolated from Foxc1 lacZ embryos has been studied [45] , the molecular mechanisms by which Foxc1 controls endochondral formation are largely unknown. Our results demonstrated that Foxc1 functionally associates with the Ihh–Gli2 signalling pathway during chondrocyte development. Because Ihh has been reported to regulate not only early chondrogenesis through the induction of PTHrP but also chondrocyte hypertrophy in a PTHrP-independent fashion [11] , [14] , our findings of Foxc1-dependent regulation of both PTHrP and Col10a1 are consistent with the multiple functions of Ihh in endochondral ossification. Gli2 is the major signalling molecule that transduces the biological function of the hedgehog family of proteins. Interestingly, similar skeletal abnormalities, including delayed endochondral ossification, defects in the vertebral column, and a reduced tibial length, were also observed in Gli2-deficient mice [17] , [49] . Importantly, we found that the loss of this functional interaction caused by a missense mutation of Foxc1 is likely to contribute to the pathogenesis of the Axenfeld–Rieger syndrome. In addition, a DN-Foxc1 diminished chondrogenic action of Ihh. Taken together, our study indicates a novel paradigm; interaction between Foxc1 and Ihh–Gli2 signalling is required for normal skeletal development ( Supplementary Fig. 13 ). Our screening system did not include a cell expansion step, which has several advantages over gene expression profiling using cultured cells. Cartilage tissues exist in unique physiological conditions that cannot be mimicked in vitro . These include a three-dimensional structure, abundant extracellular matrix, the absence of vessels and hypoxia. However, because it is generally accepted that these conditions affect chondrocyte gene expression, our screening system enables us to identify transcription factors that genuinely function in vivo . Indeed, Venus-positive cells showed high expression of Sox5 , Sox6 and Sox9 , which are known essential transcription factors involved in chondrogenesis ( Table 1 ). Moreover, several reports have indicated that the combination of tissue-specific reporter mice and FACS-assisted microarray profiling is a useful tool in gene screening. For example, Nakamura et al . [50] identified Wwp2 as a Sox9 target gene in chondrocytes using Sox9-3′ EGFP knock-in mice, while Ieda et al . [51] identified three transcription factors that enable the direct reprogramming of dermal fibroblasts into functional cardiomyocytes using the αMHC promoter. Although we focused on Foxc1 in this study, other genes identified by microarray analysis might play important roles in endochondral ossification. Although we showed that Foxc1 regulates Gli2 function by promoting DNA binding of Gli2 to target gene promoters, details of the mode of action remain to be elucidated. One possibility is that Foxc1 promotes chromatin accessibility as a pioneer factor and thereby regulates gene expression. Pioneer factors are known to open up local chromatin structure through chromatin remodelling, and many forkhead family transcription factors function as pioneer factors [52] . For example, FOXA1 is required for the optimal chromatin conditions needed for the DNA binding and gene expression induced by nuclear receptors, including oestrogen and androgen receptors [53] , [54] . Because Foxc1 does not contain a functional domain that regulates chromatin remodelling, it might recruit a variety of chromatin-modifying enzymes to regulate gene expression. It would be interesting to further investigate the transcriptional partner(s) of Foxc1 in chondrocytes during endochondral ossification. Our present results indicate that Foxc1 directly regulates PTHrP expression in chondrocytes ( Fig. 3 ). PTHrP is expressed in perichondrial cells and delays chondrocyte hypertrophy by maintaining their proliferation. Our detection of Foxc1 in perichondrial cells ( Supplementary Fig. 2a ) and in the elongated hypertrophic chondrocyte zone in the tibial growth plate of Foxc1 ch/ch mice ( Fig. 2d ) support the important role of the Foxc1–PTHrP axis during endochondral ossification. However, the skeletal phenotype of the sternum in Foxc1 ch/ch mice showing a complete absence of hypertrophic chondrocytes, is not consistent with PTHrP inhibiting chondrocyte hypertrophy. One explanation for this is that morphogenetic processes that are different between the sternum and long bones influence the phenotype differences. For example, during sternal development, bilateral sternal cartilage bars migrate towards the midline and fuse to form the sternum; this is followed by chondrocyte hypertrophy and ossification [55] , suggesting a critical role for cell migration during the development of the sternum. Interestingly, Foxc1 is expressed in the sternum primordium of the E12.5 mouse embryo [45] and several reports indicate that it is involved in the migration of various types of cells, including germ [56] , endothelial [57] and breast cancer cells [58] . These data suggest that Foxc1-dependent cell migration also contributes to skeletal development. Reduced cell migration activity could, therefore, partly account for the failure of sternum development in Foxc1 ch/ch mice ( Fig. 2b ). We found that Foxc1 is widely expressed in growth plates; therefore, it is likely that Foxc1 has multifunctional roles in several stages of cartilage development. Foxc1 ch/ch mice showed elongation of the hypertrophic chondrocyte zone ( Fig. 2c,d ), whereas the Col10-positive chondrocyte area was significantly decreased in E15.5 ( Supplementary Fig. 4c ), E17.5 ( Supplementary Fig. 8 ) and P0 Foxc1 ch/ch tibia ( Fig. 5f,g ). There is a discrepancy between these phenotypes because type-10 collagen is a well-established specific marker for hypertrophic chondrocytes. Mechanistically, we speculate that reduced Col10 expression makes hypertrophic chondrocytes functionally immature, and subsequently causes their terminal differentiation to be delayed. To support this notion, MMP13 expression was markedly decreased in Foxc1 ch/ch mice ( Fig. 2f ). The extended hypertrophic chondrocyte zone is likely due to impaired terminal differentiation, which causes inhibition of vascular invasion and subsequent replacement with bone. Further analysis is needed to characterize the hypertrophic chondrocytes observed in Foxc1 ch/ch mice. Among the forkhead protein family members, Foxc2 is most closely related to Foxc1, suggesting that the two proteins may functionally overlap. In this study, we found that Foxc2 is expressed in growth plate chondrocytes and increases PTHrP and Col10a1 expression in primary chondrocytes ( Supplementary Fig. 10 ). Foxc2-deficient mice also showed skeletal abnormalities [59] and the deletion of both Foxc1 and Foxc2 in mice resulted in early embryonic lethality [43] . However, the observed skeletal phenotype of Foxc1 ch/ch did not perfectly match that of Foxc2 -deficient mice. For instance, no cleft palate was seen in Foxc1 ch/ch mice yet this was observed in Foxc2 -deficient mice together with normal sternum development [59] . Thus, Foxc1 and Foxc2 have redundant and diverse roles in cartilage development. We also showed that the F112S mutation in the forkhead DNA-binding domain, responsible for the Axenfeld–Rieger Syndrome, causes loss of the functional association between Foxc1 and Gli2 ( Fig. 6 ). The F112S mutation leads to abnormal craniofacial development and dental abnormalities [41] ; however, the molecular basis of this is unknown. It has been reported that disease-causing missense mutations in the forkhead DNA-binding domain of FOXC1 cause various effects on the structure and function of Foxc1 (refs 29 , 60 , 61 ). For example, I91S and R127H mutations result in nuclear localization defects, while S82T, S131L and R127H mutations reduce the DNA-binding activity. Because the F112S mutation does not affect DNA binding ( Fig. 6f ), its clinical consequences are likely to result from the failure of transcriptional machinery complex formation, including the involvement of Gli2. It is possible that F112S disrupts the local protein structure, which, in turn, causes abnormal organization of the functional domain located outside the forkhead domain. Moreover, the electrostatic charge distribution on the protein surface might be altered, affecting protein–protein interactions. Molecular modelling or protein structure analysis of the F112S mutation is necessary to uncover the molecular basis of its effect. In addition to skeletal abnormalities, human FOXC1 mutations lead to dental anomalies including missing or small teeth. Interestingly, human PTHLH mutations are also reported to cause missing teeth [40] . PTHrP and the PTH/PTHrP receptor are expressed in tooth buds [62] , [63] , and overexpression of a constitutively active PTH/PTHrP receptor in mice causes a reduction in the number of ameloblasts and disorganization of the odontoblast layer [64] . These data collectively suggest that the Foxc1–PTHrP axis is also involved in tooth development, and it will be of interest to elucidate the role of Foxc1 during tooth morphogenesis to help determine the pathogenesis of the dental anomalies observed in the Axenfeld–Rieger syndrome. In conclusion, we identified a novel function for Foxc1 as a critical transcription factor for endochondral ossification. This function modulates the expression of chondrogenic genes through its physical and functional interaction with Ihh–Gli2 signalling. Our findings contribute to an improved understanding of the molecular mechanisms underlying endochondral ossification and provide new insights into the transcriptional network system of skeletal development. Generation of Col2a1 -venus transgenic mice Venus cDNA (kindly provided by Dr Atsusi Miyawaki, Lab for Cell Function Dynamics, BSI, RIKEN, Japan) was amplified by PCR and fused to the Col2a1 promoter. This transgene vector, containing a polyA site, was linearized using Not I digestion and used to generate transgenic mice by pronuclear injection. DNA was injected into single-cell BDF1 zygotes to generate transgenic mice. To determine mouse genotypes, genomic DNA isolated from tail biopsies was analysed by PCR using specific primers for Venus cDNA (sense primer: 5′-TGGTGGTGCAAATCAAAGAA-3′, antisense primer: 5′-TAGGCTTTCCACGTCGATCT-3′). All experiments were performed under protocols approved by the Osaka University Graduate School of Dentistry animal committee. Microarray analysis We dissected rib cartilage, vertebrae and limb buds from E13.5 Col2a1-Venus-Tg mice and digested the tissues into single cells using 0.1% collagenase and 0.1% trypsin. Venus-positive and Venus-negative cells were sorted with a FACS Aria flow cytometer (Becton-Dickinson, NY, USA) using the manufacturer’s instructions. Total RNA was extracted using NucleoSpin RNA II (Macherey-Nagle, Duren, Germany) without a cell expansion step. Microarray analysis was performed using the Affymetrix Mouse Genome 430 2.0 Array according to the manufacturer’s protocol (Affymetrix, Santa Clara, CA, USA). Microarray data have been deposited in NCBI Gene Expression Omnibus ( http://www.ncbi.nlm.nih.gov/geo/ ) under the accession number GSE65350 . RT–qPCR Total RNA was denatured at 65 °C for 5 min and then cDNA was synthesized using a ReverTra Ace qPCR RT Master Mix (TOYOBO, Osaka, Japan). For quantification of mRNA, RT–qPCR amplification was performed using the TaqMan PCR protocol and the ABI StepOne Plus real-time PCR system (Applied Biosystems, Foster city, CA, USA). Primers and TaqMan probes used for amplification are listed in Supplementary Table 2 . mRNA expression was normalized to that of β-actin. Data are represented as means±s.d. ( n =3). Whole-mount in situ hybridization A 594-bp fragment of Foxc1 was amplified using specific primers (sense primer: 5′-CAGAGCTCCCTCTACAGCTCC-3′, antisense primer: 5′-TCAGAATTTGCTACAGTCATA-3′) and subcloned into a pCR2 TOPO vector (Invitrogen, CA, USA). A 405-bp Col2a1 fragment subcloned into pBluescript SK vector was kindly provided by Dr Toshihisa Komori (Nagasaki University Dental School, Nagasaki, Japan). Plasmid vectors containing Foxc1 and Col2a1 fragments were linearized using BamHI (Foxc1) and EcoRI (Col2a1), respectively. Digoxigenin (DIG)-labelled antisense RNA probes for Foxc1 or Col2a1 were generated with SP6 or T7 RNA polymerase, respectively, and using a DIG RNA Labeling kit (Roche, Basel, Switzerland) according to the manufacturer’s instructions. C57BL/6 mouse embryos (E12.5) were fixed in 4% paraformaldehyde (PFA) in PBS overnight at 4 °C. Samples were hybridized overnight at 70 °C with gene-specific DIG-labelled RNA probes, then washed and incubated with anti-DIG antibody conjugated to alkaline phosphatase (anti-DIG-AP antibody, Roche) at a 1:2,500 (v/v) dilution. Nitroblue tetrazolium and 5-bromo-4-chloro-3′-indolyphosphate p-toluidine were used for signal detection. In situ hybridization Tibias from E14.5 or E15.5 mice were fixed in 4% PFA–PBS overnight at 4 °C, embedded in paraffin and cut into 5-μm sections. DIG-labelled single-stranded RNA probes were prepared using a DIG RNA labelling kit (Roche) according to the manufacturer’s instructions. The sections were deparaffinized and hybridized with chondrocyte gene-specific DIG-labelled RNA probes for 8 h at 70 °C. The signals were detected with alkaline phosphatase-conjugated anti-DIG-AP antibody at a 1:2,500 (v/v) dilution. Plasmid vectors containing fragments of Foxc1 (594 bp), Foxc2 (458 bp), Col2a1 (405 bp), Sox9 (456 bp), Ihh (579 bp), Ppr (779 bp), Col10a1 (637 bp), Col1a1 (320 bp) and Runx2 (634 bp) were linearized using Xba I (Ppr), EcoRI (Col2a1, Ihh and Col1a1), BamHI (Foxc1, Foxc2, Col10a1 and Runx2) or NcoI (Sox9), respectively. DIG-labelled antisense RNA probes were generated with SP6 (Ppr and Sox9), T3 (Col2a1, Col1a1 and Runx2) or T7 (Foxc1, Foxc2, Ihh and Col10a1) RNA polymerase using a DIG RNA Labeling kit according to the manufacturer’s instructions. These chondrocyte gene probes were kindly provided by Dr Noriyuki Tsumaki (Kyoto University, Kyoto, Japan) and Toshihisa Komori (Nagasaki University Dental School, Nagasaki, Japan). Immunohistochemical and immunofluorescence analyses Samples were fixed with 4% PFA–PBS, embedded in paraffin and cut into 4-μm-thick sections. The sections were deparaffinized and stained with Mayer’s haematoxylin and eosin. Immunohistochemistry was performed using the following antibodies: anti-Col2 (#7050; Chondrex, WA, USA) at a 1:500 (v/v) dilution, anti-MMP13 (#ab39012; Abcam, Cambridge, UK) at a 1:50 (v/v) dilution and anti-Foxc1 (#ab5079) at a 1:50 (v/v) dilution. Antigen retrieval was performed by heat mediation in a citrate buffer (pH 6) for Foxc1 and 5% hyaluronidase in PBS for 30 min at 37 °C for Col2 and MMP13. Immunoreactivity was visualized with a biotinylated anti-rabbit IgG secondary antibody using the ABC Vectastain kit (Vector Laboratories, CA, USA) and the peroxidase substrate DAB kit (Vector Laboratories), according to the manufacturer’s protocols. For immunofluorescence staining, Alexa Fluor 555-conjugated anti-rabbit IgG was used at a 1:500 (v/v) dilution as secondary antibody to visualize immunoreactivity. Counterstaining was performed using 4′,6-diamidino-2-phenylindole. Foxc1 ch/ch mice Foxc1 ch (congenital hydrocephalus, ch) heterozygous mice were purchased from the Jackson Laboratory (Bar Harbour, ME, USA) and maintained on a standard 12:12-h light/dark cycle. Homozygous Foxc1 ch/ch mice were obtained by mating heterozygous Foxc1 ch/+ mice [65] . To determine mouse genotypes, genomic DNA was amplified using a Foxc1-specific primer pair (sense primer: 5′-TATGAGCGTGTACTCGCACCCT-3′; antisense primer: 5′-CGTACCGTTCTCCGTCTTGATGTC-3′) and PCR products were then digested with Cac 8I (ref. 43 ). The WT gene yields 178 bp 197 bp fragments and the Foxc1 ch gene yields a 375 bp fragment. All experiments were performed with E15.5, E17.5 and newborn littermates under protocols approved by the Osaka University Graduate School of Dentistry animal committee. Skeletal preparation The skin of newborn and E15.5 mice was removed and fixed with 95% ethanol overnight. Cartilage tissues were stained with 1.5% Alcian blue followed by staining of bone tissues with 0.02% alizarin red. Skeletal preparation samples were photographed under a stereoscopic microscope. Cell culture and reagents HEK293, 293FT and COS-7 cells were purchased from the RIKEN Cell Bank (Tsukuba, Japan) or Life Technologies, and cultured in Dulbecco’s modified Eagle’s medium (Sigma-Aldrich, MO, USA) containing 10% fetal bovine serum at 37 °C in a humidified 5% CO 2 incubator. Isolation of primary chondrocytes Mouse primary chondrocytes were isolated according to the protocol described by Gartland et al . [66] In brief, the rib cartilage was dissected from newborn mice and digested with 0.1% collagenase D (Roche) and 0.5% trypsin (Life Technologies, CA, USA) for 6 h at 37 °C and then centrifuged for 5 min at 1,500 g . The supernatant was removed and the pellet resuspended with α-minimum essential medium containing 10% fetal bovine serum and antibiotics. Cells within two passages were used as primary chondrocytes for experiments. Construction of expression vectors and transfection WT and mutant Foxc1 cDNAs were amplified by PCR and subcloned into the Eco R I and XbaI sites of an expression vector containing 6 × Myc, Flag and 3 × Flag epitopes. The primer pairs used for PCR were as follows (WT Foxc1 : sense primer: 5′-GAATTCCAGGCGCGCTACTCGGTGTCC-3′, antisense primer: 5′-TCTAGACTAGAATTTGCTACAGTCATAGAC-3′) (DN- Foxc1 : sense primer: 5′-GAATTCGACATGGTGAAGCCGCCCTAC-3′, antisense primer: 5′-TCTAGATTAGATGCAGGGTGGTGGCTGGC-3′). RFP-tagged Foxc1 was generated by subcloning into pTurbo RFP-C (Evrogen, Moscow, Russia). DNA fragments of Gli2 and DN mutants of Gli2 (amino acids 2–497) were generated and tagged with the Myc-epitope by subcloning PCR products into pcDNA3 (ref. 67 ). Transfection of expression vectors was carried out using FuGENE6 (Roche) according to the manufacturer’s protocol. Generation of adenovirus Recombinant adenoviruses carrying Flag-tagged cDNAs of Foxc1, Flag-tagged DN-Foxc1, Flag-tagged-F112S mutant, Flag-tagged Foxc2, Myc-tagged Gli2 and Myc-tagged DN-Gli2 (ref. 67 ) was constructed by homologous recombination between the pAxCAwt expression cosmid cassette (Takara Bio, Shiga, Japan) and the parental virus genome in HEK293 cells. The viruses were confirmed to retain no proliferative activity in cells other than HEK293 cells. The expression of proteins was determined by western blotting using anti-Flag antibodies. Western blotting Cells were rinsed twice with PBS and solubilized in lysis buffer (20 mM HEPES (pH 7.4), 150 mM NaCl, 1 mM EGTA, 1.5 mM MgCl 2 , 10% glycerol, 1% Triton-X-100, 10 μg ml −1 aprotinin, 10 μg ml −1 leupeptin, 1 mM 4-(2-aminoethyl) benzenesulfonyl fluoride hydrochloride, 0.2 mM sodium orthovanadate). The lysates were centrifuged for 10 min at 4 °C at 15,000 g and boiled in SDS sample buffer containing 0.5 M β-mercaptoethanol for 5 min. Samples were then separated by SDS–polyacrylamide gel electrophoresis, transferred to nitrocellulose membranes, immunoblotted with primary antibodies and visualized with horseradish peroxidase-coupled anti-mouse (1:10,000) or -rabbit(1:5,000) immunoglobulin IgG antibodies using enhanced chemiluminescence detection kits (GE Healthcare, Buckinghamshire, UK). Anti-Flag (#F3165, 1:10,000) antibodies were purchased from Sigma-Aldrich. Anti-Myc (#ab9132, 1:2,000) was purchased from Abcam. Full scans of western blotting data are shown in Supplementary Fig. 14 . Reporter assays A firefly luciferase reporter construct containing six copies of the Foxc1 -binding element from the PTHrP promoter (5′-CAGCAGGAC TAAATAAC CAAATCCT-3′) or from the Col10a1 promoter (5′-TAAAAGTA TTTATTTAT GTGTAAGT-3′) was subcloned into pGL4.23 (Promega, WI, USA). Reporter constructs were co-transfected with Foxc1 expression vectors into COS-7 cells using FuGENE6. Forty-eight hours after transfection, the cells were lysed and luciferase activity was measured using specific substrates in a luminometer (Promega) according to the manufacturer’s protocol. IP-western analysis Cells transfected with Flag–Foxc1 and Myc–Gli2 were washed three times with ice-cold PBS and solubilized in lysis buffer. The lysates were centrifuged at 15,000 g for 20 min at 4 °C and incubated with anti-Flag M2 magnetic beads for 4 h at 4 °C. Immunoprecipitated samples were collected by a magnetic separator and washed five times with ice-cold PBS. Samples were boiled in SDS sample buffer and supernatants were subsequently subjected to western blot analysis. Confocal microscopy RFP-tagged WT or RFP-tagged F112S mutant Foxc1 were concomitantly transfected with Venus-tagged Gli2 into HEK293 cells using FuGENE 6. Forty-eight hours after transfection, the cells were fixed with 4% formaldehyde/PBS and washed three times with PBS. Samples were visualized using the Nikon A1 confocal microscope system (Nikon Instech, Tokyo, Japan). The images of x – z and y – z stacks were obtained using Nikon NIS-Elements AR software. DNA pull-down assays 293FT cells were transfected with Flag–Foxc1 and lysed using lysis buffer (20 mM HEPES (pH 7.4), 150 mM NaCl, 1 mM EGTA, 1.5 mM MgCl 2 , 10% glycerol, 1% Triton-X-100, 10 μg ml −1 leupeptin, 1 mM phenylmethanesulfonyl fluoride, 0.2 mM sodium orthovanadate), then incubated for 3 h with 1 μg of a biotinylated double-stranded oligonucleotide probe containing the Foxc1-binding element present in the PTHrP promoter (sense primer: 5′-AGCAGGACTAAATAACCAAATCCTT-3′, antisense primer: 5′-AAGGATTTGGTTATTTAGTCCTGCT-3′) or in the Col10a1 promoter (sense primer: 5′-AAAGCTCGAGAATATTGACTGAGATATGAAC-3′, antisense primer: 5′-GTTCATATCTCAGTCAATATTCTCGAGCTTT-3′). Precipitated oligonucleotides were collected using Streptavidin magnetic beads (Dynabeads My One Streptavidin T1, Invitrogen) and washed with lysis buffer. Magnetic beads were resuspended with SDS sample buffer, boiled for 5 min and subjected to western blot analysis. ChIP assays ChIP analysis was performed using a ChIP assay kit (ChIP-IT Express; Active Motif, CA, USA) according to the manufacturer’s instructions. In brief, the primary chondrocytes infected with Foxc1 or control adenovirus were washed with PBS, and the chromatin was fixed with 1% PFA. Chromatin was prepared and immunoprecipitated with 2 μg anti-Foxc1 (#ab5079) or anti-Gli2 (#ab9132) antibodies (Abcam). DNA fragments were precipitated with protein-A magnetic beads and amplified by PCR using primer pairs specific to the PTHrP promoter containing the Foxc1-binding element. Quantitative analysis of ChIP assays was performed with qPCR and relevant primer pairs are listed in Supplementary Table 2 . Statistical analysis Data were statistically analysed by Student’s t -test to compare differences between two groups. For more than two groups, we used a one-way analysis of variance or two-way analysis of variance followed by the Tukey–Kramer test. P values <0.05 were considered statistically significant. Accession codes: Microarray data have been deposited in the NCBI Gene Expression Omnibus ( http://www.ncbi.nlm.nih.gov/geo/ ) under the accession code GSE65350 . How to cite this article: Yoshida, M. et al . The transcription factor Foxc1 is necessary for Ihh–Gli2-regulated endochondral ossification. Nat. Commun . 6:6653 doi: 10.1038/ncomms7653 (2015).